FIERY1 promotes microRNA accumulation by suppressing rRNA-derived small interfering RNAs inArabidopsis Plant microRNAs (miRNAs) associate with ARGONAUTE1 (AGO1) to direct post-transcriptional gene silencing and regulate numerous biological processes. Although AGO1 predominantly binds miRNAs in vivo, it also associates with endogenous small interfering RNAs (siRNAs). It is unclear whether the miRNA/siRNA balance affects miRNA activities. Here we report that FIERY1 ( FRY1 ), which is involved in 5′−3′ RNA degradation, regulates miRNA abundance and function by suppressing the biogenesis of ribosomal RNA-derived siRNAs (risiRNAs). In mutants of FRY1 and the nuclear 5′−3′ exonuclease genes XRN2 and XRN3 , we find that a large number of 21-nt risiRNAs are generated through an endogenous siRNA biogenesis pathway. The production of risiRNAs correlates with pre-rRNA processing defects in these mutants. We also show that these risiRNAs are loaded into AGO1, causing reduced loading of miRNAs. This study reveals a previously unknown link between rRNA processing and miRNA accumulation. Small RNAs (sRNAs) serve as sequence determinants in post-transcriptional gene silencing (PTGS) in plants. The two major types of PTGS small RNAs are microRNAs (miRNAs) and small interfering RNAs (siRNAs) [1] . Like miRNAs, PTGS siRNAs are usually 21–22 nt long, but unlike miRNAs, they are derived from double-stranded precursors from transgenes, viruses, and endogenous loci, such as the TRANS-ACTING SIRNA ( TAS ) loci [1] . The machinery underlying the biogenesis and function of miRNAs and siRNAs contains shared and distinct components [2] , [3] . miRNA precursors are processed by DICER-LIKE1 (DCL1) into mature miRNAs [4] , whereas siRNAs from transgenes, viruses, and endogenous transcripts are generated by other DCLs [2] , [3] , [5] , [6] . Both miRNAs and siRNAs undergo 3′ terminal methylation by HUA ENHANCER1 (HEN1) [7] , [8] . In addition, both types of sRNAs associate with ARGONAUTE1 (AGO1) to form the functional RNA-induced silencing complex (RISC) [1] , [2] , [3] . The partial sharing of the silencing machinery imply crosstalk and potential mutual regulation between miRNAs and siRNAs. RNA quality control (RQC) suppresses siRNA production from many endogenous transcripts. Among the RQC genes are those encoding 5′-3′ EXORIBONUCLEASE3 (XRN3) and XRN4; the decapping complex subunits DECAPPING1 (DCP1), DCP2, and VARICOSE (VCS); the SUPERKILLER (SKI) complex components SKI2 and SKI3, which are involved in 3′-5′ exoribonucleolytic RNA degradation; Nonsense-mediated decay components UPFRAMESHIFT1/3 (UPF1/3); the 3′-5′ POLY(A)-SPECIFIC RIBONUCLEASE (PARN); and exosome subunits RIBOSOMAL RNA PROCESSING4 (RRP4) and RRP6L1 [1] , [9] , [10] , [11] , [12] , [13] . The sRNAs produced when these RQC genes are compromised are usually 21–22 nt long, phased, and dependent on the PTGS siRNA pathway [10] , [12] . Zhang et al. proposed that aberrant RNAs accumulated in these mutants are bound by SUPPRESSOR OF GENE SILENCING3 (SGS3) [14] and serve as templates for siRNA biogenesis [15] . Interestingly, a study on the decapping complex demonstrated that DCP1, DCP2, and VCS are required for the accumulation of some miRNAs [16] . Ribosomal RNA (rRNA)-derived sRNAs have been observed in several organisms. In Schizosaccharomyces pombe , defects in TRAMP-mediated RNA surveillance trigger the biogenesis of Ago1-associated, rRNA-derived siRNAs (rr-siRNAs) [17] . In Neurospora crassa , 20–21 nt qiRNAs are produced from aberrant rRNAs in an RdRP (RNA-dependent RNA polymerase)-dependent manner, are enriched in 5′ U, and are loaded into the AGO protein QDE-2 [18] . qiRNAs are thought to function in DNA damage repair. In Caenorhabditis elegans , 22-nt rRNA-derived siRNAs (risiRNAs) corresponding to both strands of rDNA are generated under conditions that induce pre-rRNA processing defects. C. elegans risiRNAs are enriched in 5′ G and are thought to regulate rRNA abundance [19] , [20] . In Arabidopsis , rDNA-derived 24-nt siRNAs were first described in 2006 [21] . These siRNAs are produced in a Pol IV-dependent and DCL3-dependent manner and guide DNA methylation [21] , [22] . Later studies also found 21-nt small RNAs originating from bidirectional transcripts from the intergenic spacers (IGS) of rRNA genes [23] , [24] . A recent report found that viral infections trigger the production of siRNAs from rRNAs, but the molecular or biological impacts of these ribosomal small RNAs remain unknown [25] . In this study, a mutation in FIERY1 ( FRY1 ) is isolated in a genetic screen aimed at uncovering new factors in the miRNA pathway. FRY1 encodes a dephosphorylating enzyme that converts 3′-phosphoadenosine 5′-phosphosulfate (PAPS) into adenosyl 5′-phosphosulfate (APS) in sulfur assimilation [26] , [27] . FRY1 also converts 3′-phosphoadenosine 5′-phosphate (PAP) into 5′ AMP and Pi. FRY1 functions in various biological processes, such as stress signaling [27] , drought tolerance [28] , cell elongation, flowering time [29] , leaf development [30] , root development [31] , and plant immunity [32] . fry1 mutant phenotypes resemble those of higher-order xrn mutants, possibly because accumulated PAP suppresses XRN enzymatic activity, thereby compromising 5′-3′ RNA degradation [31] , [33] , [34] . Several studies have shown that FRY1 and XRNs function in RNA degradation and suppress PTGS in Arabidopsis [9] , [33] , [35] , [36] . In a fry1 mutant, 21-nt sRNAs from the 5′ external transcribed spacer (ETS) of rRNAs accumulate in a DCL2/4-dependent manner [37] . In addition, miRNA processing intermediates accumulate in fry1 , possibly due to compromised XRN activity [9] , [38] . We find that fry1 mutations lead to the accumulation of 21–22-nt siRNAs from mRNAs and rRNAs, transcripts that do not normally undergo siRNA biogenesis. The production of risiRNAs in fry1 , as well as xrn2 xrn3 mutants correlate with pre-rRNA processing defects in these mutants. We show that the siRNAs depend on the PTGS siRNA pathway for biogenesis and are loaded into AGO proteins, AGO1 and AGO2. More importantly, risiRNAs compete with miRNAs for these AGO proteins, resulting in the compromised abundance of miRNAs. Removal of risiRNAs partially rescues both the miRNA abundance defects and the plant phenotypes of fry1 . Collectively, the findings provide insights into the biogenesis of endogenous siRNAs and the crosstalk between siRNAs and miRNAs. A mutation in FIERY1 was isolated from a suppressor screen CTR1 is a negative regulator in the ethylene response pathway [39] . ctr1 mutants exhibit constitutive ethylene responses, resulting in shorter root and hypocotyl, tightened apical hook, and swollen hypocotyl [40] . We took advantage of this conspicuous “triple” response phenotype to construct a visual reporter of miRNA activity. We designed an artificial miRNA targeting CTR1 (amiR-CTR1) driven by a β-estradiol-inducible promoter (Fig. 1a ). Upon induction, the transgenic line harboring amiR-CTR1 exhibited the ctr1 mutant phenotype (Supplementary Fig. 1a ), consistent with amiR-CTR1 accumulation and reduced CTR1 expression (Supplementary Fig. 1b, c ). This reporter line was mutagenized by EMS, and M2 plants were screened for mutants resembling wild-type (WT) plants after induction. One mutant, T5520 (Fig. 1b ), with a compromised triple response was isolated. As expected, analysis of amiR-CTR1 and CTR1 protein levels in T5520 revealed reduced accumulation of amiR-CTR1 (Fig. 1c ) and partial recovery of CTR1 protein levels (Supplementary Fig. 1d ) compared to the amiR-CTR1 parental line after β-estradiol induction. T5520 also had pleiotropic phenotypes, including round leaves and delayed flowering (Fig. 1d and Supplementary Fig. 1e ). The leaf phenotypes differed from those of canonical miRNA biogenesis mutants such as ago1 and hyl1 [41] . Fig. 1 FRY1 promotes miRNA accumulation. a A diagram of the amiR-CTR1 reporter system. Mutations that disrupt miRNA biogenesis and/or function are expected to impair the regulation of CTR1 by amiR-CTR1 and, consequently, the “triple response” phenotype. b Phenotypes of 5-day-old Arabidopsis seedlings. Upon induction, amiR-CTR1 plants exhibited the ctr1 phenotype, whereas T5520 seedlings failed to show the ctr1 phenotype. Scale bar = 5 mm. c Detection of amiR-CTR1 in T5520. Upon β-estradiol induction, amiR-CTR1 strongly accumulated in amiR-CTR1 plants. However, the accumulation was compromised in T5520 (two biological replicates separated by the red dashed line). d Phenotype of T5520 without β-estradiol induction. T5520 plants were smaller than WT and had abnormal leaves. Scale bar = 5 mm. e RNA gel blot assay for endogenous miRNAs. All four miRNAs showed reduced accumulation in fry1-6 . The U6 snRNA was used to determine the relative miRNA levels (as indicated by the numbers below the blots) between the two genotypes. Source data are provided as a Source Data file Full size image To identify the causal mutation in T5520, we conducted whole-genome re-sequencing using pooled plants with the mutant phenotypes in the F2 population of the T5520 x Col-0 cross. A G- > A mutation in AT5G63980 ( FIERY1 / SAL1 , FRY1 hereafter) was identified and verified by genotyping. The mutation was in the acceptor site of the second intron and resulted in the skipping of exon 3 and the creation of an early stop codon (Supplementary Fig. 1f–h ). Thus, T5520 is likely a null mutant of FRY1 . The FRY1 coding sequence rescued the developmental abnormalities of T5520 (Supplementary Fig. 1i ). FRY1 promotes the accumulation of miRNAs The reduced accumulation of amiR-CTR1 in T5520 suggested that the fry1 mutation impacted miRNA biogenesis. Unfortunately, the amiR-CTR1 transgene was silenced in T3 and later generations, which prevented further studies of amiR-CTR1. To determine whether FRY1 promotes miRNA accumulation, we examined endogenous miRNAs in two FRY1 T-DNA insertion lines, SALK_020882 (previously named fry1-6 [9] ) and SALK_151367 (designated as fry1-8 hereafter). RNA gel blot analysis showed that miR156, miR166, miR390, and miR398 had reduced abundance in fry1-6 (Fig. 1e ). 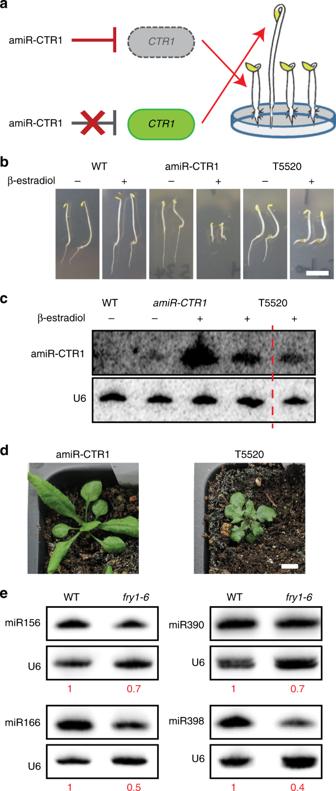Fig. 1 FRY1promotes miRNA accumulation.aA diagram of the amiR-CTR1 reporter system. Mutations that disrupt miRNA biogenesis and/or function are expected to impair the regulation ofCTR1by amiR-CTR1 and, consequently, the “triple response” phenotype.bPhenotypes of 5-day-oldArabidopsisseedlings. Upon induction, amiR-CTR1 plants exhibited thectr1phenotype, whereas T5520 seedlings failed to show thectr1phenotype. Scale bar = 5 mm.cDetection of amiR-CTR1 in T5520. Upon β-estradiol induction, amiR-CTR1 strongly accumulated in amiR-CTR1 plants. However, the accumulation was compromised in T5520 (two biological replicates separated by the red dashed line).dPhenotype of T5520 without β-estradiol induction. T5520 plants were smaller than WT and had abnormal leaves. Scale bar = 5 mm.eRNA gel blot assay for endogenous miRNAs. All four miRNAs showed reduced accumulation infry1-6. The U6 snRNA was used to determine the relative miRNA levels (as indicated by the numbers below the blots) between the two genotypes. Source data are provided as a Source Data file To assess the global effects of fry1 mutations on endogenous miRNAs, we performed sRNA sequencing of WT, fry1-6 , and fry1-8 (Supplementary Table 1 and Supplementary Fig. 2a ). A general trend of miRNA downregulation was observed in both mutants (Fig. 2a , Supplementary Fig. 2b , and Supplementary Data 1 ), consistent with the initial finding of reduced amiR-CTR1 levels in T5520. Among the statistically significant differentially expressed miRNAs, 27 and 29 miRNAs were reduced in fry1-6 and fry1-8 , respectively, which outnumbered upregulated miRNAs (Fig. 2b ). The sRNA-seq data for the abundance changes of miR156, miR166, miR390, and miR398 were similar to those detected by RNA gel blot analysis (Figs. 2c and 1e ). miR168 was among 8 upregulated miRNAs identified by sRNA-seq, and RNA gel blot analysis for miR168 showed a similar change in abundance (Fig. 2d ). Other upregulated miRNAs included two miR395 family members targeting APS genes involved in sulfur metabolism, and the upregulation of miR395 probably might have occurred in response to the altered sulfonation pathway in fry1 [29] , [42] . A previous study also reported reduced miRNA levels in fry1 mutants, but the cause of the defect was not thoroughly investigated [9] . Fig. 2 Endogenous miRNAs are reduced in fry1 mutants. a Distribution of the fold changes for all detected miRNAs in fry1-6 and fry1-8 compared to WT. The black lines in each comparison represent the canonical “box” in a boxplot with the white dot showing the median value. The “violin” shape corresponds to the density of data. P values were calculated by a one-sample two-tailed Student’s t test. The t values are −3.5885 and −3.0781, respectively, and the df values are 227 for both comparisons. b Numbers of significantly differentially expressed (DE) miRNAs in fry1 mutants compared to WT. There are a large number of downregulated miRNAs in both fry1 alleles compared to WT. c Normalized read counts of miRNAs in Fig. 1e . Sequencing results (biological replicates are shown separately) of all four downregulated miRNAs, miR156, miR166, miR390, and miR398, are consistent with those from RNA gel blot assays. d RNA gel blot validation of upregulated miR168. The left panel shows the normalized read counts from sRNA-seq. The right panel shows the RNA gel blot for miR168 in fry1-6 compared to WT. The internal control U6 snRNA was used to determine the relative levels of miR168 in the gel blot assay. Source data are provided as a Source Data file Full size image To pinpoint the miRNA biogenesis defects in fry1 mutants, we first examined the levels of endogenous pri/pre-miRNAs and the expression of major miRNA biogenesis factors by RT-qPCR and protein gel blot assays (Supplementary Fig. 2c–e ). For six miRNAs showing reduced levels in fry1-6 and miR168, which increased in abundance in fry1-6 , we quantified the corresponding pri/pre-miRNA levels. Only one (pri/pre-miR156a) had reduced accumulation, one (pri/pre-miR390b) had increased accumulation, and pri/pre-miR159b, pri/pre-miR166a, pri/pre-miR167a, pri/pre-miR168 and pri/pre-miR393b were unaffected in fry1-6 (Supplementary Fig. 2c ). Thus, the changes in pri/pre-miRNA levels did not correlate with the abundance of the mature miRNAs, indicating that the global reduction in miRNA abundance in fry1-6 could not be explained by defects in MIR gene transcription. 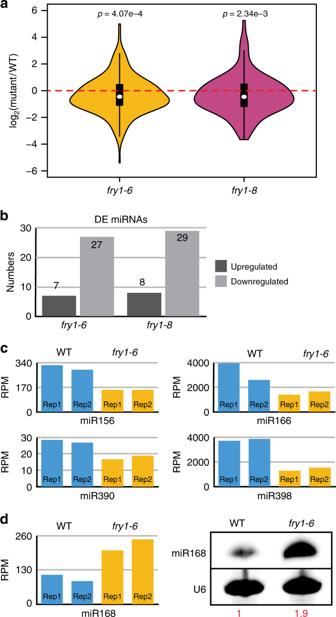Fig. 2 Endogenous miRNAs are reduced infry1mutants.aDistribution of the fold changes for all detected miRNAs infry1-6andfry1-8compared to WT. The black lines in each comparison represent the canonical “box” in a boxplot with the white dot showing the median value. The “violin” shape corresponds to the density of data.Pvalues were calculated by a one-sample two-tailed Student’sttest. Thetvalues are −3.5885 and −3.0781, respectively, and the df values are 227 for both comparisons.bNumbers of significantly differentially expressed (DE) miRNAs infry1mutants compared to WT. There are a large number of downregulated miRNAs in bothfry1alleles compared to WT.cNormalized read counts of miRNAs in Fig.1e. Sequencing results (biological replicates are shown separately) of all four downregulated miRNAs, miR156, miR166, miR390, and miR398, are consistent with those from RNA gel blot assays.dRNA gel blot validation of upregulated miR168. The left panel shows the normalized read counts from sRNA-seq. The right panel shows the RNA gel blot for miR168 infry1-6compared to WT. The internal control U6 snRNA was used to determine the relative levels of miR168 in the gel blot assay. Source data are provided as a Source Data file No substantial downregulation of the miRNA biogenesis genes was observed (Supplementary Fig. 2d ). Consistent with the increased levels of miR168 and the co-regulation of miR168 and AGO1 [43] , AGO1 protein levels were increased in both fry1 mutants (Supplementary Fig. 2e ), suggesting a compensation mechanism for reduced accumulation of miRNAs. Taken together, these results suggest that the global reduction in miRNA levels in the fry1 mutants was not due to a general defect in MIR gene transcription or pri/pre-miRNA processing. FRY1 prevents the production of ectopic siRNA To further evaluate the changes of sRNAs in fry1 at a global level, all sRNA reads in the three genotypes were mapped to the genome, and their length distribution was examined. As expected, the WT distribution was characterized by a smaller 21-nt peak and a larger 24-nt peak. In both fry1 mutants, however, the 21-nt peak was enhanced with a concomitant reduction in the 24-nt peak (Fig. 3a ), indicating an unexpected increase in 21-nt endogenous sRNAs. Fig. 3 Accumulation of 21-nt sRNAs from coding gene loci in fry1 . a Length distribution of mapped sRNA-seq reads from WT, fry1-6 , and fry1-8 seedlings. The 24-nt peak in WT nearly disappeared in both fry1 mutants. The Y axis indicates the percentage of reads of different lengths among the total mapped sRNA reads (18–42 nt). b Genomic classification of 21-nt sRNAs in WT and both fry1 mutants. See d for legends. Read counts for miRNAs decreased, and those for sRNAs from rRNAs increased dramatically in fry1-6 and fry1-8 . The annotation was adopted from known genome features. The Y axis shows the cumulative RPM values for sRNAs corresponding to different features. c Number of DSRs in fry1 mutants compared to WT. Only 21-nt and 24-nt data are shown. The 21-nt hyper DSRs greatly outnumber the other DSRs in both fry1 mutants. d Genomic classification of 21-nt hyper DSRs in both fry1 mutants. Most 21-nt hyper DSRs in fry1 corresponded to rRNA and coding genes. e Number of DSGs in fry1 mutants compared to WT. The 21-nt hyper DSGs greatly outnumber other DSGs in both fry1 mutants. f Venn diagram for genes with rogue 21-nt sRNAs in fry1-6 and fry1-8 . The overlap between the two sets is 193, which is significant based on a super exact test ( P value = 0). g Proportion of 21-nt sRNAs from 21-nt hyper DSGs among all mapped sRNA reads. The Y axis indicates the proportion of 21-nt sRNAs from the combined 21-nt hyper DSGs in both mutants (228 DSGs) among the total mapped sRNA reads. h RNA gel blot validation of rogue 21-nt sRNAs from coding genes. Two genes with abundant 21-nt siRNAs, AT1G74100 and AT3G59940, were selected. Though there are bands in WT, the signals increase in fry1-6 . i Venn diagrams for genes with rogue 21-nt sRNAs in fry1 and previously reported mutants. Except for xrn3-8 , there was a significant overlap in genes between fry1 and the analyzed mutants. See Supplementary Data 3 for details. Source data are provided as a Source Data file Full size image As the global reduction in miRNA accumulation in the fry1 mutants could not explain the increase in the 21-nt sRNA peak, we investigated changes in other categories of sRNAs. First, we examined the composition of 21-nt sRNAs. In WT, miRNAs constituted the largest category of 21-nt sRNAs in terms of abundance, with rRNA fragments being the second most abundant, followed by sRNAs from genes, TAS loci, and transposable elements (TEs). In the fry1 mutants, miRNA abundance decreased, while the abundance of sRNAs from coding genes and rRNAs increased (Fig. 3b ). Notably, rRNA fragments constituted the most abundant category of sRNAs in the mutants. To identify the sources of the differentially accumulating sRNAs, we compared sRNA abundance in 100-bp bins across the genome between fry1 and WT. Bins with higher and lower sRNA accumulation in fry1 were referred to as hyper and hypo DSRs (differential sRNA regions), respectively. We found that 21-nt hyper DSRs greatly outnumbered hyper DSRs of other lengths and hypo DSRs of all lengths in both mutants (Fig. 3c ). Many miRNA loci were among the 21-nt hypo DSRs (Supplementary Data 2 ), and the large number of 21-nt hyper DSRs was consistent with the observed increase in total 21-nt sRNAs. Genomic classification of these 21-nt hyper DSRs revealed that most of them corresponded to rRNA regions and non-miRNA genic regions, consistent with the changes in 21-nt sRNA composition (Fig. 3d ). Aberrant sRNA accumulation from coding genes Many 21-nt hyper DSRs overlapped with coding genes (Fig. 3d ). To investigate the changes in genic sRNAs, we used annotated genes as units and identified genes with differential sRNA accumulation, which we referred to as DSGs, between WT and the fry1 mutants. Hyper DSGs, i.e., genes with higher levels of sRNAs in the fry1 mutants, constituted the vast majority of DSGs (Fig. 3e ). The significant overlap in these hyper DSGs between fry1-6 and fry1-8 (Fig. 3f and Supplementary Data 3 , super exact test P value = 0) indicated that FRY1 suppresses sRNA production from these genes. There were 228 21-nt hyper DSGs in both mutants combined, and although sRNAs derived from these DSGs constituted only ~4% of the total 21-nt sRNAs (Fig. 3g , Supplementary Fig. 3a ), they represented over 10% of the total rRNA-depleted 21-nt sRNAs (Supplementary Fig. 3b ). It should be noted that most sRNA analyses in the literature ignore rRNA-derived sRNAs, which were included in this study. We selected two hyper DSGs with highly abundant sRNAs to perform RNA gel blot validation of the sRNA-seq results, and the accumulation of 21-nt sRNAs from these two genes was indeed higher in fry1-6 relative to WT (Fig. 3h ). We next investigated the possible mechanisms of sRNA accumulation from these coding genes. The accumulation of genic sRNAs was previously reported in RNA decay-deficient mutants such as ein5-1 ski2-3 , dcp2-1 , vcs , and xrn3-8 [12] , [16] , [33] . We re-analyzed the published sRNA-seq data for these mutants using our own pipeline for comparison to fry1 ( fry1-6 and fry1-8 combined). First, we examined the 21-nt hyper DSRs in these mutants and confirmed the accumulation of aberrant 21-nt sRNAs from coding genes reported in the original studies (Supplementary Fig. 3c, d ). Next, we compared 21-nt hyper DSGs between fry1 and these mutants (Fig. 3i ). The overlap between fry1 and all of the analyzed mutants was statistically significant, except for the overlap between fry1 and xrn3-8 (Supplementary Data 4 ). As XRN3 is a nuclear exonuclease while the other proteins are thought to act in cytoplasmic RNA decay, the results indicated that the aberrant genic sRNA accumulation in the fry1 mutants likely occurred in the cytoplasm. It was previously reported that in the ein5-1 ski2-3 double mutant, 21-nt sRNAs were generated from the 3′ fragments of miRNA target transcripts resulting from miRNA-guided cleavage, due to insufficient exoribonucleolytic degradation of these fragments in the cytoplasm [12] . We examined several of these experimentally validated miRNA targets with aberrant 21-nt sRNA accumulation in ein5-1 ski2-3 , but we found no accumulation of 21-nt sRNAs from these genes in fry1 (Supplementary Fig. 3e ). 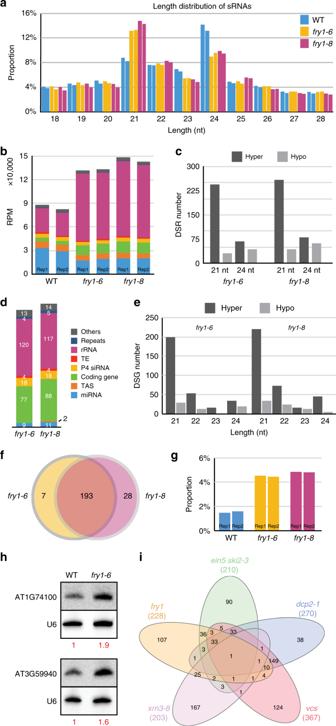Fig. 3 Accumulation of 21-nt sRNAs from coding gene loci infry1.aLength distribution of mapped sRNA-seq reads from WT,fry1-6, andfry1-8seedlings. The 24-nt peak in WT nearly disappeared in bothfry1mutants. TheYaxis indicates the percentage of reads of different lengths among the total mapped sRNA reads (18–42 nt).bGenomic classification of 21-nt sRNAs in WT and bothfry1mutants. Seedfor legends. Read counts for miRNAs decreased, and those for sRNAs from rRNAs increased dramatically infry1-6andfry1-8. The annotation was adopted from known genome features. TheYaxis shows the cumulative RPM values for sRNAs corresponding to different features.cNumber of DSRs infry1mutants compared to WT. Only 21-nt and 24-nt data are shown. The 21-nt hyper DSRs greatly outnumber the other DSRs in bothfry1mutants.dGenomic classification of 21-nt hyper DSRs in bothfry1mutants. Most 21-nt hyper DSRs infry1corresponded to rRNA and coding genes.eNumber of DSGs infry1mutants compared to WT. The 21-nt hyper DSGs greatly outnumber other DSGs in bothfry1mutants.fVenn diagram for genes with rogue 21-nt sRNAs infry1-6andfry1-8. The overlap between the two sets is 193, which is significant based on a super exact test (Pvalue = 0).gProportion of 21-nt sRNAs from 21-nt hyper DSGs among all mapped sRNA reads. TheYaxis indicates the proportion of 21-nt sRNAs from the combined 21-nt hyper DSGs in both mutants (228 DSGs) among the total mapped sRNA reads.hRNA gel blot validation of rogue 21-nt sRNAs from coding genes. Two genes with abundant 21-nt siRNAs, AT1G74100 and AT3G59940, were selected. Though there are bands in WT, the signals increase infry1-6.iVenn diagrams for genes with rogue 21-nt sRNAs infry1and previously reported mutants. Except forxrn3-8, there was a significant overlap in genes betweenfry1and the analyzed mutants. See Supplementary Data3for details. Source data are provided as a Source Data file In contrast, NIA1 and NIA2 , which are not targeted by miRNAs, generated aberrant sRNAs in fry1 (Supplementary Fig. 3e ). Moreover, only 17 of the 228 hyper DSGs in fry1 are predicted miRNA targets (Supplementary Data 5 ). We tried to identify common features of the genes that produced 21-nt sRNAs in fry1 and found that they tended to have fewer exons (Supplementary Fig. 3f ) and longer gene length, transcript length, and UTR length (Supplementary Fig. 3g–j ). Aberrant sRNA accumulation from rRNAs Besides the large number of 21-nt hyper DSRs from coding genes, over half of the 21-nt hyper DSRs were from rRNA regions. rRNA-derived sRNAs are usually considered degradation remnants of rRNAs and have typically been ignored in previous studies of sRNAs in plants. To confirm that the accumulated sRNAs arose from rRNAs and not from other overlapping features, we used the genome browser IGV [44] to visualize the detailed changes in 21-nt sRNAs at rDNA loci in all genotypes. At an rDNA locus on chromosome 3, it was obvious that regions with abundant sRNAs expanded from mature rRNA regions found in WT to the ETS/ITS (external/internal transcribed spacer) regions in fry1 (Fig. 4a ). Moreover, sRNAs were largely from the sense strand in WT, but antisense sRNAs were present in fry1 (Fig. 4a ). To verify the sRNA-seq data, we designed two probes to detect the antisense sRNAs by RNA gel blot analysis, which confirmed the accumulation of these antisense sRNAs from the rDNA locus (Fig. 4b ). This finding suggested that the sRNAs were unlikely to be rRNA degradation products. We also wondered whether rRNA-derived sRNAs similarly accumulated in the aforementioned RNA decay mutants. However, in ein5-1 ski2-3 , dcp2-1 , vcs , and xrn3-8 , no over-accumulation of sRNAs from rDNA loci (Supplementary Figs. 3d and 4a ), particularly from the ETS/ITS regions and the antisense strand (Supplementary Fig. 4b ), was observed. Although the sRNA library construction for ein5-1 ski2-3 and xrn3-8 included an rRNA removal step, rRNA fragments were still detectable due to incomplete removal. In addition, antisense rRNA fragments were not expected to have been removed by the filtering steps. Thus, the lack of ETS/ITS-derived and antisense strand-derived sRNAs suggested that the mutations in these RNA decay genes did not lead to the production of rRNA-derived sRNAs. Fig. 4 21-nt sRNAs derived from rDNA in fry1 . a An IGV view of 21-nt sRNAs mapped to an rDNA locus on Arabidopsis chromosome 3. The red and blue bars represent the normalized read counts from the positive and negative strand, respectively; all Y axis ranges in the diagram are −200 to 200. The bottom diagram shows the rDNA locus with the features indicated by black text. The red and blue text indicates the target sites of probes used in this study from the positive and negative strands, respectively. b RNA gel blot validation of antisense 21-nt sRNAs derived from rRNAs. Three biological replicates consistently show the accumulation of siRNAs corresponding to the rDNA locus in fry1-6 . The target sites of probes P6387 and P9469 are shown in a . c rRNA-derived sRNAs in xrn mutants. The rRNA-derived sRNAs were only detected in the xrn2 xrn3 mutant, but the signal intensity was still lower than that in fry1-6 . This finding suggests that the rRNA-derived sRNAs are dependent on XRN2/3. d , e Abundance of endogenous miRNAs in xrn mutants. miR166 and miR398 ( d ) were reduced in fry1-6 and to a lesser extent in xrn2 xrn3 . miR168 ( e ) increased in fry1 and xrn4 but was not affected by either the xrn2 or xrn3 mutation. Source data are provided as a Source Data file Full size image Sequence features, such as length and 5′ nucleotide identity, are highly related to Dicer processing [5] and AGO sorting [45] . We therefore examined these two features of the sRNAs that mapped to rDNA loci to determine whether they are siRNAs. As expected, sRNAs of every length (18–30 nt) arising from the sense strand were nearly equally abundant, suggesting that they correspond to rRNA degradation products. However, only 21-nt sRNAs from both strands dramatically accumulated in fry1 (Supplementary Fig. 4c ), consistent with the finding that the “rRNA” feature was enriched in 21-nt hyper DSRs but not in other size classes (Fig. 3b, c ). These findings suggested that these sRNAs might be produced by DCL1 or DCL4, which generate 21-nt sRNAs [5] . In terms of the 5′ nucleotide preference among the 21-nt sRNAs in the mutants, U was the most common 5′ nucleotide among sense sRNAs, while C was the preferred 5′ nucleotide among antisense sRNAs (Supplementary Fig. 4d ). The 5′ nucleotide preferences therefore suggested that the aberrantly accumulated sRNAs were siRNAs that loaded into AGO proteins. Defects in 5′-3′ rRNA processing lead to sRNA accumulation rRNA-derived sRNAs were observed when Arabidopsis plants were infected with viruses [25] . The production of these siRNAs depends on RDR1 , which is induced by viral infection [25] . We sought to determine the source and biogenesis requirements of rRNA-derived sRNAs in fry1 mutants. XRN2, XRN3, and FRY1 are known to be involved in rRNA processing; in xrn2 , xrn2 xrn3 , and fry1 mutants, various forms of aberrant rRNAs accumulate [37] , [46] . We therefore investigated the integrity of the rRNA processing pathway in the fry1 mutants and the relationship between aberrant rRNAs and the biogenesis of 21-nt sRNAs. For the analysis, we included the rRNA processing mutants xrn2-1 and atprmt3-2 as positive controls [46] , [47] and xrn3-2 , which exhibits normal rRNA processing, as the negative control [37] , [46] . In all of the genotypes, the abundance of mature 25S and 18S rRNAs was similar (Supplementary Fig. 5a ). Next, we used well-established probes to examine the ITS regions by RNA gel blot analysis. Consistent with previous reports, both xrn2-1 and atprmt3-2 showed changes in rRNA intermediates containing ITS sequences, while xrn3-2 did not have obvious differences compared to WT (Supplementary Fig. 5b ). Interestingly, both fry1-6 and fry1-8 had greater accumulation of 35S, 27S, and pre-5.8S rRNAs compared to xrn2-1 (Supplementary Fig. 5b ). These differences may be the consequence of defects in both XRN2 and XRN3 function in fry1 , as the accumulation of aberrant rRNAs in the xrn2 xrn3 double mutant was similar to that of fry1 mutants [37] . We also analyzed the accumulation of miRNAs and rRNA-derived sRNAs in the xrn2 , xrn3 , and xrn2 xrn3 mutants. rRNA-derived sRNAs only accumulated in fry1-6 and xrn2 xrn3 (Fig. 4c ). In addition, the abundance of miR166 and miR398 was only reduced in fry1-6 and xrn2 xrn3 (Fig. 4d ), suggesting a negative correlation between the levels of miRNAs and rRNA-derived sRNAs. Intriguingly, changes in the abundance of miRNAs and rRNA-derived sRNAs correlated with the phenotypic severity of the mutants (Supplementary Fig. 5c ). However, miR168 showed similar changes in fry1-6 and xrn4 and was not affected by mutations in XRN2 or XRN3 , suggesting that low XRN4 activity caused the increase of miR168 in fry1 (Fig. 4e ). A recent study demonstrated that defects in 3′-5′ rRNA processing induced the accumulation of antisense siRNAs from rRNA loci in C. elegans [19] . We examined the accumulation of rRNA-derived sRNAs in the Arabidopsis exosome mutant mtr4 , which exhibits defects in 3′-5′ rRNA processing and has marginal effects on PTGS [37] , [48] . Using the same probes, however, we could not detect any sRNAs from the analyzed rDNA locus in the mtr4 mutant (Supplementary Fig. 5d ). These findings indicated that the biogenesis of 21-nt sRNAs from aberrant rRNAs in Arabidopsis resulted specifically from defects in 5′-3′ exonuclease activity. Rogue 21-nt sRNAs are products of the PTGS pathway To further investigate whether the coding-gene-derived and rRNA-derived sRNAs were siRNAs, we examined whether their biogenesis required RDR and/or DCL proteins. We crossed fry1-6 with known siRNA biogenesis mutants, including rdr1-1 , rdr2-1 , rdr6-11 , dcl2-1 , dcl3-1 , and dcl4-2 [49] , [50] , [51] . Intriguingly, the biogenesis of coding-gene-derived sRNAs and rRNA-derived sRNAs was different. The accumulation of rRNA-derived antisense sRNAs in fry1-6 was completely suppressed by rdr6-11 , weakly affected by rdr2-1 and unaffected by rdr1-1 (Fig. 5a ). Meanwhile, although 21-nt rRNA-derived sRNAs were eliminated in fry1-6 dcl4-2 , sRNAs of predominantly 22 nt accumulated from the same loci (Fig. 5a ). This was due to DCL2, as in the fry1-6 dcl2-1 dcl4-2 triple mutant, 21–22-nt sRNAs were almost gone (Fig. 5a ). However, for coding-gene-derived sRNAs, RDR1 was crucial for their biogenesis as rdr1-1 suppressed the enhanced sRNA accumulation in fry1-6 (Fig. 5b ). Moreover, these sRNAs accumulated even more in the fry1-6 rdr6-11 mutant than in fry1-6 , which might be the consequence of the slightly upregulated RDR1 expression in the absence of RDR6 function (Supplementary Fig. 6a ). Similar to rRNA-derived sRNAs, dcl2-1 and dcl4-2 together completely suppressed the over accumulation of coding-gene-derived sRNAs (Fig. 5b ). Fig. 5 Rogue 21-nt sRNAs are dependent on RDR s and DCL s for biogenesis. a Accumulation of rRNA-derived sRNAs in rdr and dcl mutants as determined by RNA gel blot assays. For the antisense sRNAs corresponding to the rDNA locus, rdr6-11 has a suppressive effect, while rdr2-1 has only a minor suppressive effect. dcl4-2 enhances the accumulation of longer sRNAs from these two loci, while in fry1-6 dcl2-1 dcl4-2 , no accumulation of 21-nt or 22-nt siRNAs was detected. This indicated the antagonistic roles of DCL2 and DCL4 in siRNA biogenesis at these loci. b RNA gel blot assays to determine the abundance of coding-gene-derived sRNAs in rdr and dcl mutants. Unlike rRNA-derived sRNAs, these sRNAs largely depend on RDR1 for biogenesis. Besides, both DCL2 and DCL4 are required for the accumulation of coding-gene-derived sRNAs. Black arrows indicate the 21-nt sRNAs. c , d Regions generating phased siRNAs in WT and fry1 . At TAS genes TAS1A and TAS3 ( c ), phasing scores were slightly reduced in fry1 . However, there are many phased regions from rDNA detected only in fry1 ( d ). Source data are provided as a Source Data file Full size image As the biogenesis of these 21-nt rogue sRNAs required RDR1 / 6 and DCL2 / 4 , we concluded that these sRNAs were siRNAs and, more specifically, ribosomal siRNAs (risiRNAs) for the rRNA-derived ones. The biogenesis requirements of these rogue siRNAs are similar to those of another class of endogenous siRNAs, namely phasiRNAs, which exhibit a head-to-tail phasing signature [3] . Hence, we next investigated the phasing of rogue siRNAs using established methods [52] . Surprisingly, the phasing scores at TAS and genes known to generate phasiRNAs were slightly reduced in the two fry1 mutants, while those at the rDNA locus and many 21-nt hyper DSGs were drastically increased (Fig. 5b–d , Supplementary Fig. 6b ). These findings reinforced the conclusion that rogue siRNAs, including risiRNAs, were produced from double-stranded RNAs by processive DCL activity. 21-nt risiRNAs are loaded into AGO1 To address whether the 21-nt risiRNAs had any biological impacts in vivo, we first examined whether these siRNAs are loaded into AGO1 by immunoprecipitation (IP) of AGO1 in WT and fry1-6 (Supplementary Fig. 7a ), followed by sequencing of the sRNAs from the IP products (Supplementary Data 6 ). Three independent experiments were performed. As expected, 21-nt sRNAs were enriched and 24-nt sRNAs were depleted in the AGO1 IP sRNA-seq (Fig. 6a ). In addition, 5′ U was a predominant feature of sRNAs in both IP products (Supplementary Fig. 7b ). This indicated that AGO1 IP sRNA-seq was successful. Fig. 6 Association of 21-nt risiRNAs with AGO1. a Length distribution of mapped reads from sRNA-seq of AGO1 IP in WT and fry1-6 . The proportion of 21-nt reads in all mapped reads is slightly higher in fry1-6 than in WT. b Genomic classification of 100-bp bins with an enrichment of 21-nt sRNAs in AGO1 IP vs. input from WT and fry1-6 . Although the numbers of bins corresponding to miRNAs and ta-siRNAs are similar between WT and fry1-6 , those of bins corresponding to coding genes and rRNAs dramatically increased in fry1-6 . The annotation was adopted from known genome features. c Distribution of 5′ nucleotides among 21-nt sRNAs derived from rRNA regions. In WT, a 5′-U preference was only observed among reads from the antisense strand in AGO1 IP, while in fry1-6 , a 5′-U preference was observed among reads from both strands. This discovery suggests that the majority of sense reads in WT are not bound by AGO1, while those in fry1-6 can be loaded into AGO1. d Venn diagrams for genes with enriched 21-nt sRNAs. In AGO1 IP, most genes with enriched 21-nt sRNAs identified in WT were also identified in fry1-6 . The 1224 genes in fry1-6 also included most of the 21-nt hyper DSGs identified in fry1 . Source data are provided as a Source Data file Full size image As a preliminary analysis, we used the genome browser to examine AGO1 binding of risiRNAs. At the rDNA locus on chromosome 3, 21-nt sRNAs were depleted in AGO1 IP from WT but enriched on both strands, including the ETS/ITS regions, in AGO1 IP from fry1-6 (Supplementary Fig. 7c ). We then conducted IP enrichment analysis in WT and fry1-6 : IP-enriched bins were defined as 100-bp bins with a statistically significant increase in sRNA abundance in IP versus input. In WT, most enriched bins were from miRNA and other genes, including TAS genes, and there were only 7 enriched bins from rRNA regions (Fig. 6b ). Compared to WT, the numbers of enriched bins from miRNA and TAS genes were similar, but the number of enriched bins from rRNA regions increased in fry1-6 (Fig. 6b ). We also examined the 5′ nucleotides of these risiRNAs (Fig. 6c ). In WT, 5′-U sRNAs constituted about 40% of sense and over 80% of antisense 21-nt sRNAs associated with AGO1. In fry1-6 , the 5′-U percentages were over 90 and 80% for sense and antisense 21-nt sRNAs, respectively. These findings suggested that in WT, many of these sense sRNAs might not be loaded into AGO1 despite their association with it, whereas rogue rRNA-derived sRNAs from both strands in fry1-6 could be loaded. Notably, there were also more 21-nt sRNAs and more enriched 21-nt bins from coding genes in fry1-6 (Fig. 6b ). Therefore, we conducted a similar IP enrichment analysis for genes and identified 193 and 1224 genes as those enriched for AGO1-associated 21-nt sRNAs in WT and fry1-6 , respectively (Fig. 6d ). As expected, the 1224 genes in fry1-6 included most of the 193 genes identified in WT. The 1224 genes also included most of the 228 hyper DSGs identified in fry1 . Interestingly, the low overlap between the 228 hyper DSGs (i.e., genes with rogue 21-nt sRNAs in fry1-6 and fry1-8 ) and the 193 genes with AGO1-bound 21-nt sRNAs in WT suggested that the genes suppressed by FRY1 for sRNA production were distinct from those that generated sRNAs in WT. We also analyzed the sequence features of the 1224 IP-enriched genes in fry1-6 , and the results supported the hypothesis that longer genes with fewer exons tended to generate 21-nt siRNAs in fry1 (Supplementary Fig. 7d–h ). The loading of miRNAs into AGO1 is compromised in fry1-6 Because most miRNAs associate with AGO1 under normal conditions, the miRNA-binding capacity of AGO1 might be compromised by the excessive accumulation of risiRNAs and siRNAs from other coding genes in fry1 . To support the hypothesis that rogue siRNAs compete with miRNAs for loading into AGO1, we conducted small RNA-seq following AGO1 IP in fry1-6 rdr6-11 , in which risiRNAs were barely detectable (Fig. 5a ) (Supplementary Table 1 and Supplementary Data 6 ). As expected, around 50% of the 21-nt sRNAs associated with AGO1 were derived from rRNA in fry1-6 , while the corresponding proportion in WT was less than 5%, according to the genomic classification of AGO1-associated 21-nt sRNAs (Fig. 7a ). Consistent with results from the RNA gel blot assay (Fig. 5a ), the proportion of risiRNAs in AGO1 was substantially reduced in fry1-6 rdr6-11 (Fig. 7a and Supplementary Fig. 8a ). In addition, the fraction of AGO1-associated miRNAs decreased to less than 30% in fry1-6 , and was restored to over 50% by the rdr6-11 mutation (Fig. 7a ). Although the numbers of enriched miRNAs in AGO1 IP were similar in WT, fry1-6 (Fig. 6b ), and fry1-6 rdr6-11 (Supplementary Fig. 8b ), the loading efficiency of miRNAs, as represented by the ratio of miRNA levels in IP and input, was slightly decreased in fry1-6 and restored in fry1-6 rdr6-11 (Supplementary Fig. 8c, d and Supplementary Data 7 ). Specifically, for the 20 most abundant miRNAs in WT, the IP/input ratios were significantly reduced in fry1-6 (Fig. 7b and Supplementary Fig. 8e , paired Wilcoxon test P value = 0.001718) and recovered in fry1-6 rdr6-11 (paired Wilcoxon test P value = 0.003654 between fry1-6 rdr6-11 and fry1-6 ). These results indicated that in fry1-6 AGO1′s binding to miRNAs declined, and AGO1 associated with risiRNAs. The reduced miRNA abundance in fry1 mutants was likely due to the compromised loading of miRNAs into AGO1. Fig. 7 r dr6-11 partially rescues the fry1 phenotypes. a Genomic classification of 21-nt AGO1-associated sRNAs. In WT, miRNAs and ta-siRNAs constitute the majority of AGO1-associated 21-nt sRNAs. In fry1-6 , there is a drastic increase in rRNA-derived siRNAs, consistent with the total sRNA composition. The rdr6 mutation results in a partial removal of risiRNAs and a concomitant partial restoration of miRNAs. The Y axis shows the cumulative RPM values for sRNAs corresponding to different genomic features. b The AGO1 loading efficiency of the 20 most abundant miRNAs in WT. The loading efficiency is represented by the ratio of RPM in immunoprecipitated samples to that in input. The efficiencies in WT and fry1-6 are significantly different based on a paired Wilcoxon test ( P value = 0.001718). The efficiencies are recovered by the rdr6 mutation ( fry1-6 rdr6-11 vs. fry1-6 : P value = 0.003654; fry1-6 rdr6-11 vs. WT: P value = 0.114). c , d miRNA accumulation in rdr and dcl mutants. miR166 and miR398 are downregulated in fry1-6 , and all three analyzed double mutants show slightly higher abundance of the miRNAs than fry1-6 ( c ). However, the increased abundance of miR168 in fry1-6 was still present in the double mutants ( d ). The internal control U6 snRNA was used to determine the relative miRNA levels. e Partial rescue of the fry1 phenotypes by rdr and dcl mutations. Plants shown are at 22 days after germination. rdr6-11 can partially rescue the mutant phenotypes of fry1-6 . Meanwhile, DCL4 is necessary for the survival of fry1 mutants, probably due to the enhanced activity of DCL2 in dcl4-2 . This was supported by the fry1-6 dcl2-1 dcl4-2 triple mutant. The restoration of leaf shape by rdr6-11 is shown by the enlarged leaves in the insets. Source data are provided as a Source Data file Full size image To further support the above hypothesis, we examined the abundance of miRNAs in mutants whose risiRNAs were suppressed or partially suppressed, including fry1-6 rdr2-1 , fry1-6 rdr6-11 , and fry1-6 dcl4-2 . In all these mutants, the downregulation of miR166 and miR398 was partially suppressed (Fig. 7c ). However, the upregulation of miR168 was not affected in any of these double mutants compared to fry1-6 (Fig. 7d ). Furthermore, the rdr6-11 mutation partially restored the fry1 mutant phenotype, especially the leaf shape phenotype (Fig. 7e ). However, dcl4-2 did not rescue the fry1 phenotype, and the fry1-6 dcl4-2 double mutants were extremely small and died at about 22 days after germination (DAG) (Fig. 7e ). This was similar to the phenotype of the ein5-1 ski2-3 dcl4 triple mutant, in which enhanced biogenesis of 22-nt siRNAs from endogenous genes by DCL2 led to further production of secondary siRNAs [12] . However, while dcl2 dcl4 can fully rescue the ein5-1 ski2-3 mutant phenotype [12] , the phenotype of the fry1-6 dcl2-1 dcl4-2 triple mutant was similar to that of fry1-6 but not WT (Fig. 7e ). This also suggested that the developmental phenotypes of fry1 were not fully attributable to rogue siRNAs. Because rogue siRNAs were loaded into AGO1, we sequenced the transcriptome of WT, fry1-6 , fry1-6 rdr6-11 , and fry1-6 rdr1-1 to understand if the siRNAs affected gene expression. Despite the large numbers of upregulated and downregulated genes (Supplementary Fig. 8f, g ), we focused on known miRNA targets and the 200 genes generating siRNAs in fry1-6 (Fig. 3f ). Among 10 representatives of known miRNA targets, 7 of them showed upregulated expression in fry1-6 , and this upregulation was reduced in at least one of the fry1-6 rdr6-11 and fry1-6 rdr1-1 mutants (Supplementary Fig. 8h ). This suggested that mutations in either RDR6 or RDR1 can partially restore miRNA activity in the fry1 mutant. 186 genes accumulating siRNAs in fry1-6 were detectably expressed by the RNA-seq and they showed different expression patterns in fry1-6 rdr1-1 and fry1-6 rdr6-11 . In fry1-6 rdr1-1 , where siRNA biogenesis from these genes was compromised, the expression of these genes was upregulated significantly as compared to WT. Congruously, their expression decreased in fry1-6 rdr6-11 , in which siRNA biogenesis from these genes was enhanced (Supplementary Fig. 8i ). This indicated that either siRNA biogenesis would eliminate transcripts from these genes or accumulated siRNAs would target the corresponding transcripts for cleavage. The loading of miRNAs into AGO2 is compromised in fry1-6 We noticed that miR390, which is predominantly bound by AGO7 and AGO2 [53] , also decreased in abundance in fry1-6 (Fig. 1e and Fig. 2c ). This may also be attributed to compromised loading of miR390 into AGO2/7 due to competition from rogue siRNAs. Thus, we tested the loading of AGO2-associated miRNAs by AGO2 IP followed by sRNA sequencing in WT, fry1-6 , and fry1-6 rdr6-11 (Supplementary Data 6 ). The composition of 21-nt reads, the most abundant length in AGO2 IP samples (Supplementary Fig. 9a ), was very different among the three genotypes. In WT, AGO2 mainly associated with miRNAs and trans-acting siRNAs (ta-siRNAs), while in fry1-6 risiRNAs and coding-gene-derived siRNAs constituted the majority of AGO2-associated sRNAs (Supplementary Fig. 9b ). Meanwhile, as rdr6-11 removed ta-siRNAs and a portion of risiRNAs, the proportion of AGO2-associated miRNAs increased in fry1-6 rdr6-11 compared to the fry1-6 single mutant (Supplementary Fig. 9b ). Next, we conducted analyses to identify genomic regions showing statistically higher levels of sRNAs in AGO2 IP relative to input. In fry1-6 , the number of enriched bins corresponding to coding genes and Pol IV-dependent siRNA regions drastically decreased while that of rRNA bins increased as compared to WT (Supplementary Fig. 9c ). Consistent with the findings from AGO1 IP (Fig. 6b and Supplementary Fig. 8b ), the fry1-6 rdr6-11 mutant also showed a partial restoration of AGO2′s sRNA binding profile in terms of the numbers of enriched bins (Supplementary Fig. 9c ). We specifically examined known AGO2-bound miRNAs [53] , including miR159, miR390, and miR408 (Supplementary Data 8 ). The levels of the miRNAs in AGO2 IP decreased in fry1-6 but were slightly restored in fry1-6 rdr6-11 (Supplementary Fig. 9d ). 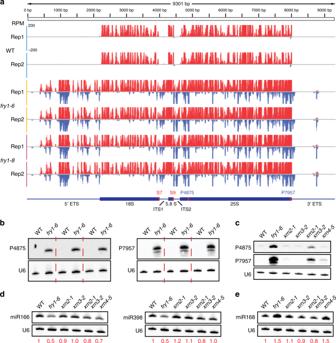Fig. 4 21-nt sRNAs derived from rDNA infry1.aAn IGV view of 21-nt sRNAs mapped to an rDNA locus onArabidopsischromosome 3. The red and blue bars represent the normalized read counts from the positive and negative strand, respectively; allYaxis ranges in the diagram are −200 to 200. The bottom diagram shows the rDNA locus with the features indicated by black text. The red and blue text indicates the target sites of probes used in this study from the positive and negative strands, respectively.bRNA gel blot validation of antisense 21-nt sRNAs derived from rRNAs. Three biological replicates consistently show the accumulation of siRNAs corresponding to the rDNA locus infry1-6. The target sites of probes P6387 and P9469 are shown ina.crRNA-derived sRNAs inxrnmutants. The rRNA-derived sRNAs were only detected in thexrn2 xrn3mutant, but the signal intensity was still lower than that infry1-6. This finding suggests that the rRNA-derived sRNAs are dependent on XRN2/3.d,eAbundance of endogenous miRNAs inxrnmutants. miR166 and miR398 (d) were reduced infry1-6and to a lesser extent inxrn2 xrn3. miR168 (e) increased infry1andxrn4but was not affected by either thexrn2orxrn3mutation. Source data are provided as a Source Data file We then examined the coding gene-derived siRNAs and risiRNAs. 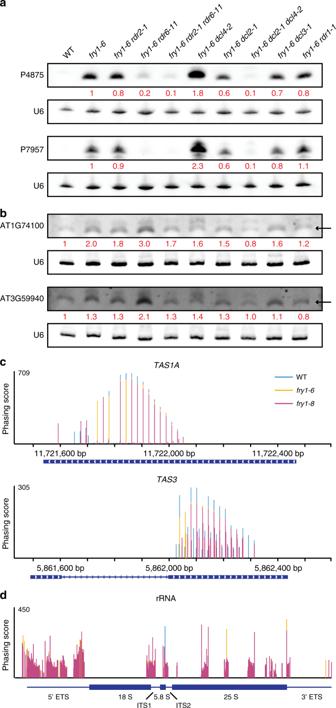Fig. 5 Rogue 21-nt sRNAs are dependent onRDRs andDCLs for biogenesis.aAccumulation of rRNA-derived sRNAs inrdranddclmutants as determined by RNA gel blot assays. For the antisense sRNAs corresponding to the rDNA locus,rdr6-11has a suppressive effect, whilerdr2-1has only a minor suppressive effect.dcl4-2enhances the accumulation of longer sRNAs from these two loci, while infry1-6 dcl2-1 dcl4-2, no accumulation of 21-nt or 22-nt siRNAs was detected. This indicated the antagonistic roles ofDCL2andDCL4in siRNA biogenesis at these loci.bRNA gel blot assays to determine the abundance of coding-gene-derived sRNAs inrdranddclmutants. Unlike rRNA-derived sRNAs, these sRNAs largely depend onRDR1for biogenesis. Besides, bothDCL2andDCL4are required for the accumulation of coding-gene-derived sRNAs. Black arrows indicate the 21-nt sRNAs.c,dRegions generating phased siRNAs in WT andfry1. AtTASgenesTAS1AandTAS3(c), phasing scores were slightly reduced infry1. However, there are many phased regions from rDNA detected only infry1(d). Source data are provided as a Source Data file AGO2 bound siRNAs from 154 of the 228 genes with rogue siRNAs in fry1 (Supplementary Fig. 9e ). Also, 5′ A, which is preferred by AGO2 [45] , was enriched in risiRNAs from both strands (Supplementary Fig. 9f ). We noticed that, although rdr6-11 suppressed the loading of risiRNAs into AGO2, there were still 80 bins of risiRNAs in fry1-6 rdr6-11 (Supplementary Fig. 9c, g ), and most of them were from the 5′ ETS (Supplementary Fig. 9g ). These results suggested that the loading of sRNAs into AGO2 was affected in fry1-6 . Because sRNAs from rDNA regions are usually considered degradation products of mature rRNAs, many previous sRNA-seq analyses have often excluded these sequences by removing them during library construction or after read mapping during data analysis. Still, some studies have reported the existence of rRNA-derived siRNAs and implicated their functions. In S. pombe , because rr-siRNAs preferentially begin with 5′ U and associate with Ago1, they may sequester Ago1 and interfere with its function [17] . Recent studies in C. elegans have described similar phenomena: under conditions such as 3′-5′ exonuclease impairment, cold stress, and deficient rRNA processing, 22-nt siRNAs with a 5′-G preference accumulated from both strands of rDNA. These risiRNAs can be loaded into NRDE-3, a nuclear Ago protein, and potentially target rRNA precursors [19] , [20] . In Arabidopsis , 24-nt siRNAs from rDNA involved in the RNA-directed DNA methylation pathway was first identified [21] , [22] . These siRNAs are not derived from rRNA precursors or mature rRNAs as they are generated in a Pol IV-dependent manner. Small RNAs generated from rRNAs or their precursors have also been found in plants. Some vasiRNAs in virus-infected Arabidopsis are from rRNAs, are 21-nt long, and are dependent on DCL4 and RDR1 for biogenesis [25] . Similarly, rRNA-derived 21-nt siRNAs accumulate in xrn2 xrn3 and fry1 mutants [37] . But neither of these reports provided evidence for the AGO association of these rRNA-derived small RNAs. In this study, we report the extreme accumulation of AGO1-associated and AGO2-associated risiRNAs in plants. We showed that sRNAs arose from both strands and from the EST/IST regions of the rDNA loci in fry1 (Fig. 4b ) and that they competed with miRNAs for loading into AGO1 and AGO2. Since the accumulation of risiRNAs was dependent on XRN2/3 (Fig. 4c ), it is reasonable to assume that their biogenesis occurs in the nucleus. Nuclear risiRNAs would pose a threat to miRNAs, which are loaded into AGO1 in the nucleus [54] . On the other hand, the present findings indicate that risiRNA biogenesis is also dependent on RDR6 and DCL4 (Fig. 5a ), which localize to both the cytoplasm and the nucleus [55] , [56] , [57] , complicating predictions about the site of risiRNA biogenesis. Based on the present findings, we propose a competition model as shown in Fig. 8 . In WT plants, FRY1 degrades PAP to ensure the activities of XRN4 in the cytoplasm and XRN2/3 in the nucleus. XRN4 and XRN2/3 efficiently degrade aberrant RNAs in the cytoplasm and nucleus, respectively, which prevents the biogenesis of siRNAs. Thus, most AGO1 proteins are occupied by miRNAs. In the fry1 mutants, PAP accumulates and inhibits the activity of XRNs. Aberrant mRNAs and rRNAs accumulate and are captured by the siRNA pathway, which consequently generates rogue siRNAs that compete with miRNAs to occupy AGO1 and AGO2 proteins. Perhaps as an attempt to reach miRNA homeostasis, AGO1 levels were increased in fry1 (Supplementary Fig. 2e ) [43] . However, excessive risiRNAs and siRNAs from coding genes still outcompeted miRNAs, resulting in their low loading efficiency and reduced abundance. Thus, the proper partitioning of AGO1 for miRNA and siRNA binding requires RQC. Fig. 8 A proposed model of FRY1 function in balancing siRNA and miRNA biogenesis in Arabidopsis . In WT plants (upper half of the diagram), FRY1 degrades PAP to ensure the activation of XRN2/3/4 function. XRNs degrade aberrant RNAs to prevent the biogenesis of rogue siRNAs. As a result, most AGO (AGO1 and AGO2) proteins are associated with miRNAs and function in miRNA-directed target regulation. In fry1 mutants (lower half of the diagram), PAP accumulates and inhibits XRN activity. The resulting aberrant RNAs, including mRNAs and rRNAs, are captured by the PTGS siRNA pathway. Rogue 21-nt sRNAs are generated from the aberrant RNAs by RDR1 and RDR6, respectively, and compete with miRNAs for AGO occupancy. The altered partitioning of AGO between miRNAs and siRNAs leads to reduced abundance of miRNAs Full size image Consistent with previous findings in cytoplasmic RNA decay mutants [12] , the fry1-6 dcl4-2 double mutant was not viable but viability could be restored by the dcl2-1 mutation (Fig. 7e ). Nevertheless, the fry1-6 dcl4-2 dcl2-1 triple mutant, like fry1-6 rdr2-1 and fry1-6 rdr6-11 , still exhibited abnormal phenotypes compared to WT plants (Fig. 7e ), indicating only a partial rescue of fry1 by mutations in the siRNA pathway. Indeed, the abundance of miR166 and miR398 was only partially restored in fry1-6 rdr6-11 that lacked rogue siRNAs (Fig. 7c ). FRY1 and XRN2/3 facilitate the turnover of excised pre-miRNA loops in Arabidopsis [9] . This defect in miRNA processing may also affect the abundance of mature miRNAs. The partial rescue of fry1 by rdr6-11 or dcl2-1 dcl4-2 differs from the full phenotypic rescue of ein5-1 ski2-3 by the same mutations [12] , but resembles the minimal rescue of dcp2-1 and vcs-6 by rdr6 sgs2-1 10 . We also noticed that there were still abundant risiRNAs from the 5′ ETS in all rdr6 samples (Supplementary Fig. S8a and 9g ); the biogenesis of these risiRNAs was RDR6 -independent. These 21-nt risiRNAs may have originated from the bidirectional transcription of rDNA, as previously reported [23] and may account for the partial rescue of fry1 phenotypes by rdr6 . Despite this, the fry1 mutant phenotypes may not be entirely attributable to the accumulation of risiRNAs and 21-nt siRNAs from coding genes. Other processes affected in fry1 , such as RNA processing, RNA decay, and sulfur metabolism, may also contribute to the phenotypes. In summary, we show that RNA silencing activity is impacted by competition between miRNAs and siRNAs for AGO1 in Arabidopsis , and RNA quality control maintains small RNA homeostasis to ensure proper miRNA activities. Plant materials and growth Arabidopsis thaliana wild-type (accession Columbia-0) and T-DNA insertion lines of FRY1 (AT5G63980, fry1-6 : SALK_020882, fry1-8 : SALK_151367), XRN2 (AT5G42540, xrn2-1 : SALK_041148), XRN3 (AT1G75660, xrn3-2 : SAIL_762H09), XRN4 (AT1G54490, xrn4-5 : SAIL_681E01), PRMT3 (AT3G12270, atprmt3-2 : WISCDSLOX391A01), RDR1 (AT1G14790, rdr1-1 : SAIL_672F11), RDR2 (AT4G11130, rdr2-1 : SAIL_1277H08), RDR6 (AT3G49500, rdr6-11 : CS24285), DCL2 (AT3G03300, dcl2-1 : SALK_064627), DCL3 (AT3G43920, dcl3-1 : SALK_005512), and DCL4 (AT5G20320, dcl4-2 : GABI_160G05) were used in this study. Seeds were germinated on 1/2 MS medium under short-day conditions (8 h light and 16 h dark) at 22 °C, and seedlings were either collected for analyses or transferred to soil for phenotypic observation on day 12. EMS mutagenesis and mutant identification amiR-CTR1 (CGGGUUGGGAAUAAUAUGUAU) was designed using WMD tools ( http://wmd3.weigelworld.org/cgi-bin/webapp.cgi ) then inserted into the MIR319a backbone [58] . The amiR-CTR1 fragment was recombined into the plasmid pER10 containing a β-estradiol-induction cassette using the Xho1 and Spe1 restriction sites (Supplementary Data 9 ). The construct was transformed into WT Arabidopsis by Agrobacterium transformation. To locate the T-DNA insertion site, we re-sequenced the amiR-CTR1 transgenic plants on the HiSeq 2000 platform at the genomics core facility at UCR. By mapping the resulting reads to the Araport11 Arabidopsis thaliana genome ( https://www.araport.org ), we determined that the insertion was between nucleotides 18214427 and 18214448 on chromosome 5. We also confirmed that there was only a single T-DNA insertion in the genome, as no chimeric reads from two T-DNA borders (LB/RB) were found. About 2 mL freshly collected amiR-CTR1 seeds were used for ethyl methanesulfonate (EMS) mutagenesis. Seeds were washed in 0.1% Tween-20 for 15 min then treated with 50 mL 0.1% EMS overnight on a rotator in a fume hood. The seeds were transferred to 0.5 M NaOH and incubated overnight, rinsed with ddH 2 O several times, then washed in ddH 2 O for 4 h. Finally, the seeds were sown in soil. 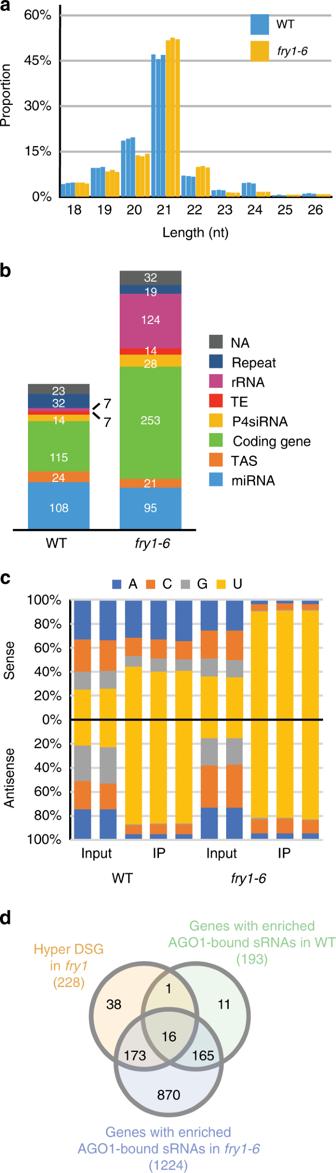Fig. 6 Association of 21-nt risiRNAs with AGO1.aLength distribution of mapped reads from sRNA-seq of AGO1 IP in WT andfry1-6. The proportion of 21-nt reads in all mapped reads is slightly higher infry1-6than in WT.bGenomic classification of 100-bp bins with an enrichment of 21-nt sRNAs in AGO1 IP vs. input from WT andfry1-6. Although the numbers of bins corresponding to miRNAs and ta-siRNAs are similar between WT andfry1-6, those of bins corresponding to coding genes and rRNAs dramatically increased infry1-6. The annotation was adopted from known genome features.cDistribution of 5′ nucleotides among 21-nt sRNAs derived from rRNA regions. In WT, a 5′-U preference was only observed among reads from the antisense strand in AGO1 IP, while infry1-6, a 5′-U preference was observed among reads from both strands. This discovery suggests that the majority of sense reads in WT are not bound by AGO1, while those infry1-6can be loaded into AGO1.dVenn diagrams for genes with enriched 21-nt sRNAs. In AGO1 IP, most genes with enriched 21-nt sRNAs identified in WT were also identified infry1-6. The 1224 genes infry1-6also included most of the 21-nt hyper DSGs identified infry1. Source data are provided as a Source Data file To find the causal mutation in T5520, the CTAB method was used to extract DNA from ~50 plants with the T5520 phenotype from the F2 population of the T5520 x Col-0 cross. A DNA library was constructed with the NEBNext Ultra™ II DNA Library Prep Kit for Illumina (E7645S, NEB) according to the manual. The library was sequenced on the HiSeq 2000 platform at the genomics core facility at UCR, and the PE150 reads were mapped to the Arabidopsis genome. SNPs were called using SAMtools v1.9 [59] then analyzed to identify the causal mutation using an online software NGM ( http://bar.utoronto.ca/ngm/index.html ). From the NGM result, we narrowed the location of the mutation to a region consisting of 10 candidate genes (AT5G49770, AT5G52170, AT5G54330, AT5G55330, AT5G57060, AT5G62770, AT5G63450, AT5G63980, AT5G64390, and AT5G64430) that contained SNPs with discordant chastity scores over 0.95. We designed dCAPS primers for all of the candidate genes and analyzed another batch of F2 plants with the mutant phenotype [60] . This analysis pinpointed the mutation to AT5G64390 ( FRY1 ). RNA extraction and northern blotting Total RNA was extracted from 12-day-old WT and mutant seedlings using TRI reagent (MRC, TR118) according to the manufacturer’s instructions. For each sample, 10 μg total RNA was run on a 15% urea-PAGE gel and transferred to a Hybond NX membrane. The RNA was cross-linked to the membrane with the EDC cross linking buffer (0.16 M EDC, 0.13 M 1-methylimidazole at pH 8.0) at 65 °C for 90 min. Biotin-labeled probes were added to the hybridization buffer (5X SSC, 20 mM Na 2 HPO 4 at pH 7.2, 7% SDS, 2× Denhardt’s solution) and incubated with the membrane at 55 °C overnight. After two wash steps (2X SSC, 0.1%SDS, 55 °C, 20 min each time) to remove excess probe, the membrane was processed using the Chemiluminescent Nucleic Acid Detection Module Kit (ThermoFisher, 89880) according to the instruction manual with probes described in Supplementary Data 9 . The relative expression level in the RNA gel blots was calculated against the internal control U6 using Fiji [61] . Protein detection Aerial tissues (25 mg) of 12-day-old seedlings were harvested for protein extraction using 1× SDS buffer (100 mM Tris at pH6.8, 4% SDS, 20% Glycerol, 0.2% Bromophenol blue). The samples were loaded onto a 10% SDS-PAGE gel and proteins were then transferred to a nitrocellulose membrane after electrophoresis. Anti-AGO1 antibody (1:3,000, Agrisera, AS09 527) was used to detect the AGO1 protein, and the 60S ribosomal protein L13 was detected with its antibody (1:2,500, Agrisera, AS13 2650) and served as the internal control. sRNA library construction and sequencing Total RNA (20 μg) from WT (Col-0), fry1-6 , and fry1-8 was resolved on a 15% urea-PAGE gel, and the sRNA fraction (15–40 nt) was excised. sRNAs in the excised gel were recovered in 0.4 M NaCl, followed by ethanol precipitation. sRNA libraries were constructed using the NEBNext Small RNA Library Prep Set for Illumina (NEB, E7300S) according to the manufacturer’s instructions. The libraries were pooled and sequenced to generate 75-bp single-end reads on an Illumina NextSeq CN500 platform at Berry Genomics (Beijing, China). Analysis of sRNA-seq data Our sRNA-seq data and published datasets ( GSE57936 , GSE65056 , GSE95473 ) were analyzed using a publicly available pipeline, pRNASeqTools v0.6. The sRNA-seq raw reads were trimmed to remove the 3′ adapter sequences (AGATCGGAAGAGC) then size-selected (18–42 nt) using cutadapt v1.9.1 [62] . The trimmed reads were mapped to the Araport11 genome using ShortStack v3.4 [63] with parameters ‘-bowtie_m 1000-ranmax 50-mmap u-mismatches 0′. To calculate and compare sRNA abundance in the WT and mutant libraries, the Arabidopsis genome was tiled into 100-bp bins (or bins based on specific features, e.g., miRNAs, TEs, genes, and 1000-bp gene-upstream sequences), and reads whose 5′ end nucleotides mapped to a given bin were assigned to that particular bin. Normalization was conducted by calculating the RPM value ( r eads p er m illion mapped reads) for each bin, and comparison was performed for each category of bins using the R package DESeq2 [64] . The significance of overlap was calculated using the R package SuperExactTest [65] . sRNA target prediction was performed by psRNATarget [66] using the 2017 scheme with expectation ≤2. AGO IP and sRNA-seq Total protein was extracted from WT, fry1-6 , and fry1-6 rdr6-11 seedlings using IP buffer (50 mM Tris 7.5, 150 mM NaCl, 10% glycerol, 0.1% NP-40, and 1× proteinase inhibitor cocktail). AGO1 antibody (8 μL/g) or AGO2 antibody (16 μL/g, Agrisera, AS13 2682) and protein A Dynabeads (Invitrogen, 10002D) were sequentially added to the supernatant to obtain the AGO protein complex. For WT, fry1-6 , and fry1-6 rdr6-11 , the immunoprecipitation, RNA extraction, library construction, sequencing, and data analysis were performed in three independent experiments as described above for total sRNAs. mRNA-seq and data analysis RNA-seq libraries were constructed using NEBNext® Ultra™ RNA Library Prep Kit for Illumina® (NEB, USA) following manufacturer’s recommendations, and pooled and sequenced on the Illumina NovaSeq 6000 system (paired-end, 150 bp) at Berry Genomics (Beijing, China). The RNA-seq data were analyzed using the pRNASeqTools. 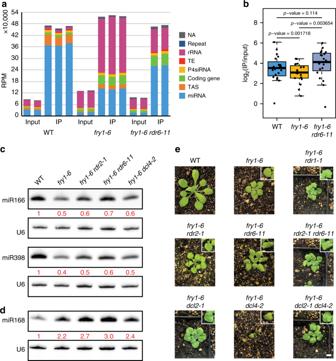Fig. 7 rdr6-11partially rescues thefry1phenotypes.aGenomic classification of 21-nt AGO1-associated sRNAs. In WT, miRNAs and ta-siRNAs constitute the majority of AGO1-associated 21-nt sRNAs. Infry1-6, there is a drastic increase in rRNA-derived siRNAs, consistent with the total sRNA composition. Therdr6mutation results in a partial removal of risiRNAs and a concomitant partial restoration of miRNAs. TheYaxis shows the cumulative RPM values for sRNAs corresponding to different genomic features.bThe AGO1 loading efficiency of the 20 most abundant miRNAs in WT. The loading efficiency is represented by the ratio of RPM in immunoprecipitated samples to that in input. The efficiencies in WT andfry1-6are significantly different based on a paired Wilcoxon test (Pvalue = 0.001718). The efficiencies are recovered by therdr6mutation (fry1-6 rdr6-11vs.fry1-6:Pvalue = 0.003654;fry1-6 rdr6-11vs. WT:Pvalue = 0.114).c,dmiRNA accumulation inrdranddclmutants. miR166 and miR398 are downregulated infry1-6, and all three analyzed double mutants show slightly higher abundance of the miRNAs thanfry1-6(c). However, the increased abundance of miR168 infry1-6was still present in the double mutants (d). The internal control U6 snRNA was used to determine the relative miRNA levels.ePartial rescue of thefry1phenotypes byrdranddclmutations. Plants shown are at 22 days after germination.rdr6-11can partially rescue the mutant phenotypes offry1-6. Meanwhile,DCL4is necessary for the survival offry1mutants, probably due to the enhanced activity of DCL2 indcl4-2. This was supported by thefry1-6 dcl2-1 dcl4-2triple mutant. The restoration of leaf shape byrdr6-11is shown by the enlarged leaves in the insets. Source data are provided as a Source Data file 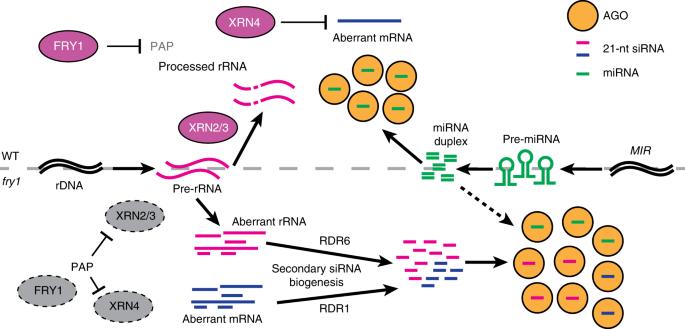Fig. 8 A proposed model ofFRY1function in balancing siRNA and miRNA biogenesis inArabidopsis. In WT plants (upper half of the diagram), FRY1 degrades PAP to ensure the activation of XRN2/3/4 function. XRNs degrade aberrant RNAs to prevent the biogenesis of rogue siRNAs. As a result, most AGO (AGO1 and AGO2) proteins are associated with miRNAs and function in miRNA-directed target regulation. Infry1mutants (lower half of the diagram), PAP accumulates and inhibits XRN activity. The resulting aberrant RNAs, including mRNAs and rRNAs, are captured by the PTGS siRNA pathway. Rogue 21-nt sRNAs are generated from the aberrant RNAs by RDR1 and RDR6, respectively, and compete with miRNAs for AGO occupancy. The altered partitioning of AGO between miRNAs and siRNAs leads to reduced abundance of miRNAs Briefly, raw reads were mapped to the Araport11 genome using STAR v2.6 [67] with the parameters “--alignIntronMax 5000 --outSAMmultNmax 1 --outFilterMultimapNmax 50 --outFilterMismatchNoverLmax 0.1”. Mapped reads were counted by featureCounts v1.6.4 [68] and comparison was performed using the R package DESeq2 [64] . Reporting summary Further information on research design is available in the Nature Research Reporting Summary linked to this article.